The overlapping burden of the three leading causes of disability and death in sub-Saharan African children 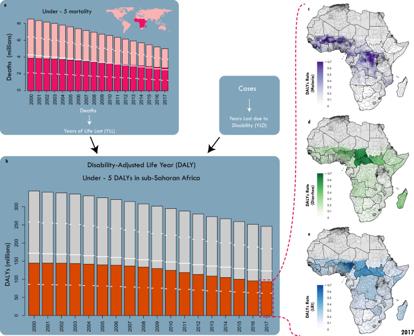Fig. 1: Global and continental trends in under-5 mortality and DALYs. aGlobal under-5 mortality from 2000 to 2017. Fuchsia indicates the fraction of those deaths that occur in sub-Saharan Africa.bTotal under-5 DALYs in sub-Saharan Africa from 2000 to 2017. Orange indicates the fraction of those DALYs attributable to the combined burden of lower respiratory infections (LRIs), diarrhoea, and malaria; Total DALYs per child: estimates of burden attributable to malaria (c, purple), diarrhoea (d, green), LRIs (e, blue), and all other causes (grey) are summed to give total DALY rates for 2017. In all panels, white dashes indicate 25th% and 75thpercentiles, and white lines indicate 50%. Maps were produced using ArcGIS Desktop 10.6. Despite substantial declines since 2000, lower respiratory infections (LRIs), diarrhoeal diseases, and malaria remain among the leading causes of nonfatal and fatal disease burden for children under 5 years of age (under 5), primarily in sub-Saharan Africa (SSA). The spatial burden of each of these diseases has been estimated subnationally across SSA, yet no prior analyses have examined the pattern of their combined burden. Here we synthesise subnational estimates of the burden of LRIs, diarrhoea, and malaria in children under-5 from 2000 to 2017 for 43 sub-Saharan countries. Some units faced a relatively equal burden from each of the three diseases, while others had one or two dominant sources of unit-level burden, with no consistent pattern geographically across the entire subcontinent. Using a subnational counterfactual analysis, we show that nearly 300 million DALYs could have been averted since 2000 by raising all units to their national average. Our findings are directly relevant for decision-makers in determining which and targeting where the most appropriate interventions are for increasing child survival. More than half of the estimated five million children under the age of 5 (under-5) who died worldwide in 2017 were from sub-Saharan Africa (SSA) (Fig. 1 ) with substantial between- and within-country variation in these mortality rates across the region [1] . The three most dominant causes of under 5 mortality in SSA in 2017—lower respiratory infections (LRIs), diarrhoeal diseases, and malaria—were responsible for 1,066,000 (95% Uncertainty Interval (UI) 807,000–1,419,000) of these deaths [2] , accounting for more than a third (39% (35–44%)) of all child mortality in SSA in that year [3] . In addition to years of life lost (YLLs), sub-Saharan African children were estimated to have a combined nonfatal disease burden of more than 9.6 million (8.1–11.4) years lived with disability (YLDs) in 2017 from these three causes [4] . The total all-cause disease burden for children in SSA from the sum of YLLs and YLDs was 245.6 million (230.7–263.1) disability-adjusted life years (DALYs) in 2017 [5] , of which over 93.2 million (70.7–124.0; 38%) were due to just these three diseases (Fig. 1 ). Each of these three dominant causes are largely preventable and treatable and thus represent a potentially avoidable disease burden. The goal of ending preventable child deaths – a primary component of Sustainable Development Goal 3.2 [6] – would be supported by identifying and reducing geographical inequality in the distribution of mortality and total disease burden for these three primary drivers at the 2 nd administrative level [1] (e.g., ‘counties’ in Kenya or ‘local government areas’ in Nigeria, hereinafter referred to as ‘units’). This second administrative level is often the implementation unit for intervention planning and delivery. Fig. 1: Global and continental trends in under-5 mortality and DALYs. a Global under-5 mortality from 2000 to 2017. Fuchsia indicates the fraction of those deaths that occur in sub-Saharan Africa. b Total under-5 DALYs in sub-Saharan Africa from 2000 to 2017. Orange indicates the fraction of those DALYs attributable to the combined burden of lower respiratory infections (LRIs), diarrhoea, and malaria; Total DALYs per child: estimates of burden attributable to malaria ( c , purple), diarrhoea ( d , green), LRIs ( e , blue), and all other causes (grey) are summed to give total DALY rates for 2017. In all panels, white dashes indicate 25 th % and 75 th percentiles, and white lines indicate 50%. Maps were produced using ArcGIS Desktop 10.6. Full size image Previous efforts to map all-cause under-5 mortality patterns have identified areas with persistently high mortality rates [1] . To act on these findings, cause-specific maps of both mortality and total disease burden (DALYs) would be beneficial for all major causes of under-5 mortality to guide specific and/or integrated intervention planning. Further, efforts to co-map individual causes simultaneously can pinpoint locations where total burden remains high despite individual cause reductions, as well as identify which disease is contributing most substantially to the disease burden in any one location. Precision public health efforts of this kind can also serve as an aid in the prioritisation of traditionally vertical public health interventions [7] and could identify opportunities for increasing delivery efficiency. For example, improvements in vaccination require microplanning of subnational efforts to ensure all children are immunised [8] , which in turn relies on knowing which locations are most in need. Using high-resolution estimates of the co-occurring and proportional disease burden from these dominant causes of child burden is thus a key step towards delivering on the promise of precision public health [9] , [10] . Disease-specific hotspots in death and disability have been previously identified across Africa for each of the three dominant causes of under-5 disease burden separately [11] , [12] , [13] . The analyses illustrate an inconsistent overlap in the geographic units with the highest disease burden from the three causes collectively in 2017 (Fig. 1a-c ). Contributing risk factors include a lack of adequate antimalarials and/or insecticide-treated bed nets (ITNs) [14] , child growth failure (CGF) [15] , micronutrient deficiency [16] , poor water quality [17] , inadequate sanitation and hygiene [18] , [19] , exposure to household air pollution [20] , and poor vaccine coverage [21] . While some risk factors, such as CGF and micronutrient deficiencies, education, and poor access to health systems, have a wide influence across many causes [22] , others, such as vaccines or ITNs, are cause-specific. Individual disease maps can be used for targeting intervention campaigns, but they do not help account for the potential efficiencies gained from taking a more systematic approach by considering multiple diseases and their underlying social or health causes simultaneously, which is often a necessity for health programs in resource-limited settings. Critically, however, hotspots for each disease do not always overlap, and as such, no single suite of interventions across diseases will optimally reduce childhood burden throughout SSA. Health loss from both nonfatal and fatal disease burden as measured in DALYs is a widely used measure of population health that captures additional health losses beyond mortality [23] (Fig. 1 ). Given infectious disease DALY burden is predominantly due to years of life lost (YLLs), disease burden estimates will closely reflect deaths due to these diseases. While the burden of each of these three causes has been individually assessed at fine spatial scales in SSA [11] , [12] , [24] , there remains no comprehensive evaluation of the overlapping burden across the subcontinent or within countries. Here we evaluate patterns in the combined burden of DALYs from LRIs, diarrhoeal diseases, and malaria (hereinafter referred to as ‘combined DALYs’ or ‘combined burden’) and assess changes in those patterns over time for children in 43 countries in SSA. We synthesised the most recent estimates, geospatially resolved to the second administrative unit level, of nonfatal and fatal disease burden for each of these three causes [11] , [12] , [13] . We calculated the combined DALYs from LRIs, diarrhoeal diseases, and malaria by summing across causes within each unit. We then conducted a counterfactual analysis comparing median disease-specific burden between subnational units within each country. By using each country’s median burden in each year as a local (nationally specific) benchmark, we show for the first time the potential impact of reducing subnational heterogeneity by improving health outcomes for those most vulnerable among these three causes on childhood survival. Understanding simultaneous trends in disease burden across these three diseases at the unit level can help local decision-makers direct resources to maximise the impact of health interventions on under-5 mortality and morbidity overall. Patterns of combined burden in 2017 Patterns of total DALYs The average total DALY rate among children across all causes of disease (all-cause DALY rate) in all sub-Saharan African countries in 2017 was 1.5 DALYs per child per year (95% uncertainty interval (UI) 1.5–1.6), accounting for 248.8 million (233.8–266.2) total all-cause DALYs (Fig. 1 ) [5] . While this burden can be decomposed into infectious and non-communicable diseases as well as injuries, more than half of it was due to infectious diseases (54.7%; 136.0 million (125.1–147.1) DALYs) [5] . Despite having proven and effective interventions [25] , LRIs, diarrhoeal diseases, and malaria were associated with about two-thirds of infectious disease burden in SSA (94.1 million (84.1–105.5); 69.2%: (64.2–74.3%)) and were responsible for more than a third of the burden among all causes in 2017 (37.8% of all DALYs [34.6–41.4%]). Nigeria, Democratic Republic of the Congo (DRC), and Ethiopia each had more than five million combined DALYs for children due to these three causes, with Nigeria accumulating over 31.4 million (20.6–45.3) combined DALYs in 2017. In terms of combined DALY rate, country-level estimates in Central African Republic (CAR), Chad, Niger, and Sierra Leone all exceeded one DALY per child per year. These countries have the highest DALY rate for children under-5 among all countries globally (the global average DALY rate for LRI, diarrhoea, and malaria was about 0.2 per child-year) [5] . Sixteen countries in SSA had average combined DALY rates above 0.5 per child-year. We used these cut-offs to indicate high (>0.5 DALY per child-year) and very high (>1 DALY per child-year) combined burden. Triple DALYs Burden As expected, there is a clear pattern where countries with a higher total all-cause burden proportionally had more of that burden attributable to LRIs, diarrhoea, and malaria combined [26] (Supplementaryy Information Fig. 1 ). Thus, at the country scale, there is a strong suggestion that general interventions that would reduce LRI, diarrhoea, and malaria burden simultaneously would have a massive impact in the countries that have the highest total all-cause childhood disease burden. The distribution of combined DALYs for LRIs, diarrhoea, and malaria exhibits substantial variation between and, importantly, within countries (Fig. 2a ). Using mean estimates, eleven countries had at least one unit whose combined mean DALY rate exceed 1 per child per year (Nigeria (297/775 units, 45% of children under-5), CAR (51/51, 100%), Chad (47/55, 89%), DRC (25/213, 6%), Burkina Faso (23/45, 42%), Niger (19/36, 65%), Mali (12/49, 28%), Sierra Leone (9/14, 67%), South Sudan (7/45, 30%), Guinea (2/34, 3%), and Benin (1/64, 2%)). Using the bounds of each country’s 95% uncertainty interval on DALYs by unit, we find that as many as 19 and as few as 2 countries may have at least one unit with a combined DALY rate greater than 1 per child. Emphasising the subnational variation, Benin, DRC, Mali, and Nigeria each also had units where the mean estimated combined rate of DALYs was less than 0.5 per child per year. Over half of all sub-Saharan countries included in this analysis (24 of 43) had at least one unit where the mean combined DALY rate was greater than 0.5 per child per year (Fig. 2a ), and among these, 19 had subnational variation large enough that some units had at least twice the mean burden of others. The CAR was anomalous in that not only did every unit in the country have an estimated mean combined DALY rate greater than one, but the relative variation (e.g., deviation divided by country average) in the country was low across all countries in SSA. Fig. 2: Combined disability-adjusted life years (DALYs) in 2017 and decomposition. a Second administrative level estimates of combined DALYs. b For second administrative units where the combined DALYs per child per year exceeded 0.5 in 2017, the primary component of the local composition of burden is plotted. Units where the combined DALYs were less than 0.5 are plotted as white. Units with dark purple have greater than 60% of their combined burden attributable to malaria (e.g., areas of Burkina Faso). Units with dark blue have greater than 60% of their combined burden attributable to LRIs (e.g., areas of Nigeria). Units with dark green have greater than 60% of their combined burden attributable to diarrhoea (e.g., areas of Chad). Units coloured light purple, blue, or green have between 50% and 60% of their combined burden attributable to malaria, LRIs, or diarrhoea, respectively. Units coloured yellow have no dominant cause (no cause’s contribution exceeds 50%). Units which are shaded dark brown have all causes represented in their combined burden with percentages between 20% and 40%. Three examples from Western sub-Saharan Africa are highlighted. For each region, the composition of the relative contribution of each cause translates to a point in the ternary plot legend. The closer a point is to each corner, the higher the relative contribution of that cause. Maps were produced using ArcGIS Desktop 10.6. Full size image Variation in primary cause Many of the countries that contained subnational units with high combined burden were the same as those that had high country-level burden for each of the three individual causes. Subnationally, there is no single consistent pattern of which cause or causes contribute the largest share to the combined burden in 2017 (Fig. 2 ). Among units with high combined burden (rate of over 0.5 DALYs per child per year as presented in colour in Fig. 2b ), some were dominated by a single cause. For example, targeting malaria in the dark purple units in Fig. 2b (such as Gourma, Est , Burkina Faso; 66.2% of the combined burden [48.7–80.2%]) or LRIs in the dark blue units in Fig. 2b (such as Adavi, Kogi , Nigeria; 52.8% of the combined burden [38.1–66.5%]) might have the largest impact in reducing under-5 DALY burden in those locations. Conversely, there were 13 countries with units with high mean combined burden of LRIs, diarrhoea, and malaria (rate > 0.5 DALYs), yet each cause made an equivalent contribution (between 20% and 40%) to that combined burden. We show these as brown units in Fig. 2b . An example is Gogounou, Alibori , Benin (malaria 37.8% [11.6–57.6%], diarrhoea 29.6% [18.0–49.0%], LRIs 32.6% [19.2–46.9%]). These units likely require more universal approaches to burden reduction. While the intensity of combined burden at the second administrative level and at the national level often coincided, such as in CAR, which had the highest country-level mean combined DALY rate (1.4 per child-year [0.9–1.9]) and two of the top 10 highest unit-level combined rates, this was not universal. Locations with high levels of combined LRI, diarrhoea, and malaria burden (Fig. 2a ) were not necessarily regionally remarkable in their burden for any single cause (Supplementary Information Tables 1 – 4 ). For example, the Gombe Shani region of Nigeria had the second-highest combined rate of DALYs in Africa in 2017, but ranked 38th, 294th, and 45 th for burden due to LRIs, diarrhoea, and malaria, respectively. Moreover, although Nigeria did not have the highest mean combined DALY rate in Africa in 2017, units within this country had the second-highest and fourth-highest mean combined DALY rates ( Yobe Shani had 1.78 [0.19–2.9] DALYs per child per year, and Bayo, Gombe had 1.76 [0.18–3.0] DALYs per child per year). This exemplifies considerable subnational variation in Nigeria (Supplementary Information Fig. 2 ). Thus, drawing conclusions on which causes are of most importance (and therefore which interventions are likely optimal) based on national-level statistics can profoundly deviate from conclusions drawn by looking specifically at the subnational units with the highest burden. Lower respiratory infections were the second leading cause of DALYs globally in SSA among children under-5 in 2017 (after neonatal disorders) and were ubiquitous across SSA. At least 29.6% (18.0–49.0) of the combined DALYs burden in every unit in SSA was attributable to LRIs, which had a population-weighted average contribution of 40.4% (20.3–65.6) of combined DALYs (Supplementary Information Fig. 2 ). In 2017, LRIs resulted in the greatest total burden of the three causes for children in SSA, but surprisingly they rarely dominated the proportional combined burden in any unit (Fig. 2b ). Among the total burden of LRIs, a majority of DALYs occurred in units where LRIs were responsible for just 19.7% (6.9–39.7) of the combined burden occurred (blue regions of Fig. 2b ). Only 5.6% (1.6–15.9) of the LRI burden occurred in a unit where LRIs resulted in more than 60% of the combined burden (dark blue regions of Fig. 2b ). As such, while LRI is the dominant cause of childhood disease burden in very few units, almost every unit would benefit from including some additional measure of LRI prevention and treatment within their combined intervention strategy. Temporal trends 2000 to 2017 Trends of combined burden also varied substantially between and within countries from 2000 to 2017. In brief, combined LRI, diarrhoea, and malaria disease burden decreased from 2000 to 2017 in almost every unit. Some of the countries with the highest combined burden, such as Niger and Sierra Leone, achieved substantial reductions but via very different pathways (Supplementary Information Fig. 2 ). Units across Niger reduced both their LRI (56.4% reduction (35.8–71.6)) and diarrhoea burden (64.0% reduction (53.8–72.9)), while their malaria burden did not change significantly over the period (31.2% increase (−23.2–133.6)). Niger introduced the Hib, pneumococcal, and rotavirus childhood vaccines between 2000 and 2017 and had important reductions in childhood growth failure, risk factors that may not have reduced the malaria disease burden [27] , [28] . In spite of the uneven trends, the current composition of combined burden across most units of Niger remains mostly equally split across the three causes (33.3% malaria (5.2–49.8), 36.6% diarrhoea (27.7–59.8), 30.2% LRIs (22.4–42.8)) (yellow and brown units in Fig. 2b ). Sierra Leone on the other hand, was more consistent in burden reduction across all three causes (27.0% malaria reduction (4.8–44.2), 63.1% diarrhoea reduction (58.0–66.6), 56.1% LRI reduction (44.1–61.2)), possibly due to large reductions in micronutrient (vitamin A and zinc) deficiency [27] . Further, in 2010, Sierra Leone introduced a government program intended to improve access to healthcare (Free Health Care Initiative) which has improved access to and equity for maternal and child health services [29] , [30] . Although rare, there were instances where disease burden in a unit increased for one of the three causes. There were however a few units where the burden from one of the dominant three diseases increased by so much that it resulted in an overall combined burden increase, most notably Zimbabwe and CAR (Supplementary Information Fig. 3 ). For units in Zimbabwe, although combined burden is slightly higher in 2017 (0.32 DALYs per child (0.22–0.46)) than 2000 (0.31 DALYs per child (0.21–0.42)), it does appear to have been declining for the past decade (after steep increases in diarrhoea burden between 2000 and 2010, a period of unrest [27] and a cholera epidemic in 2009). Conversely, there are units within CAR where increases have occurred for multiple causes. Since the combined burden in every unit of CAR is high but evenly distributed across all three causes (yellow units in Fig. 2b ), national strategy must embrace interventions to reduce all three causes simultaneously. Health conditions in CAR are dire [31] . The country has been embroiled in conflict and civil war for much of the period 2000 to 2017 and the country urgently needs improvements in basic public health measures like childhood nutrition, insecticide-treated bed nets, and childhood vaccines. Counterfactual analysis of averted burden As described above, there is subnational variation in the combined burden, its composition, and its change over time across all countries of sub-Saharan Africa. However, there are clearly some countries with generally higher combined burden and others with generally lower combined burden. Comparing units across countries, to the best-performing unit across the entire continent, would unrealistically assume the ability to achieve reductions far greater than those observed within a country. A more nationally feasible and pragmatic approach is to compare each unit to the median across units within that country and year. Accordingly, for each country for each year, we identified the median LRI burden, diarrhoea burden, and malaria burden and used these as a target benchmark for all other units in that country in that year. Since 2000, there have been an estimated 2.3 billion (2.1–2.5) combined DALYs for children in sub-Saharan Africa due to these three diseases. If every unit in every country had uniformly achieved at least the median burden levels for each disease in its respective country in each year, almost 300 million DALYs (77–743), or about 13% of that burden, could have been averted from 2000 to 2017. In 2017 alone, units performing worse than their country’s median burdens for the three diseases combined was responsible for 15.1 million (4.2–38.5) combined DALYs in SSA children (Supplementary Information Table 4 ). Based on this analysis, several units, particularly in Nigeria and DRC, could have averted a high combined DALY rate in 2017 had they performed at the level of the national median for each of the three diseases in 2017 (Fig. 3a ). Fig. 3: Counterfactual analysis in 2017. a Second administrative level reductions in combined DALY rates b Map of second administrative units in Nigeria whose averted combined DALYs exceeded 10,000, the primary component of the local composition of burden is plotted. 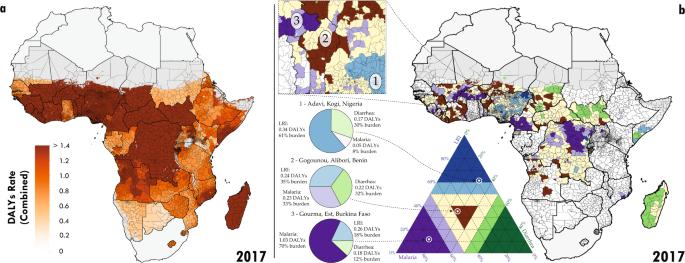Fig. 2: Combined disability-adjusted life years (DALYs) in 2017 and decomposition. aSecond administrative level estimates of combined DALYs.bFor second administrative units where the combined DALYs per child per year exceeded 0.5 in 2017, the primary component of the local composition of burden is plotted. Units where the combined DALYs were less than 0.5 are plotted as white. Units with dark purple have greater than 60% of their combined burden attributable to malaria (e.g., areas of Burkina Faso). Units with dark blue have greater than 60% of their combined burden attributable to LRIs (e.g., areas of Nigeria). Units with dark green have greater than 60% of their combined burden attributable to diarrhoea (e.g., areas of Chad). Units coloured light purple, blue, or green have between 50% and 60% of their combined burden attributable to malaria, LRIs, or diarrhoea, respectively. Units coloured yellow have no dominant cause (no cause’s contribution exceeds 50%). Units which are shaded dark brown have all causes represented in their combined burden with percentages between 20% and 40%. Three examples from Western sub-Saharan Africa are highlighted. For each region, the composition of the relative contribution of each cause translates to a point in the ternary plot legend. The closer a point is to each corner, the higher the relative contribution of that cause. Maps were produced using ArcGIS Desktop 10.6. 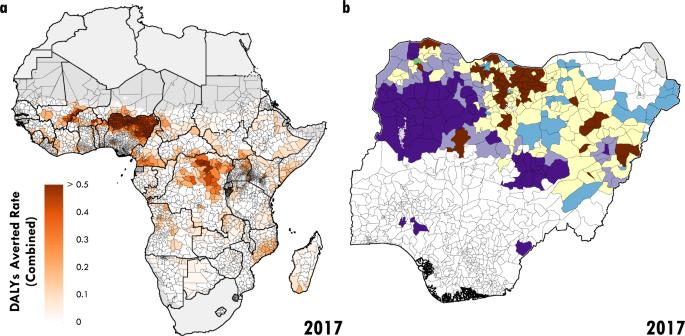Fig. 3: Counterfactual analysis in 2017. aSecond administrative level reductions in combined DALY ratesbMap of second administrative units in Nigeria whose averted combined DALYs exceeded 10,000, the primary component of the local composition of burden is plotted. Units where the combined DALYs averted were less than 10,000 are plotted as white. Units with dark purple have greater than 60% of their averted combined burden attributable to malaria. Units coloured light purple or blue have between 50% and 60% of their averted combined burden attributable to malaria or LRIs, respectively. Units coloured yellow have no dominant cause (no cause’s contribution exceeds 50%). Units which are shaded dark brown have all causes represented in their averted combined burden with percentages between 20% and 40%. Maps were produced using ArcGIS Desktop 10.6. Units where the combined DALYs averted were less than 10,000 are plotted as white. Units with dark purple have greater than 60% of their averted combined burden attributable to malaria. Units coloured light purple or blue have between 50% and 60% of their averted combined burden attributable to malaria or LRIs, respectively. Units coloured yellow have no dominant cause (no cause’s contribution exceeds 50%). Units which are shaded dark brown have all causes represented in their averted combined burden with percentages between 20% and 40%. Maps were produced using ArcGIS Desktop 10.6. Full size image More informatively, we see that in countries such as Nigeria, units that could have averted more than 10,000 DALYs over the study period (shown in colour, Fig. 3b , units averting <10,000 DALYs shown in white) would have needed to improve their performance differentially by individual disease. Indeed, the theoretical gains identified by this counterfactual analysis would not be observed uniformly across sub-Saharan Africa, and the sources for these gains vary from country to country and unit to unit. By identifying units where a specific disease has an outsized burden compared to the rest of that country (resulting in a large number of DALYs averted over the study period, shown for example as dark purple units in Fig. 3b for malaria in Nigeria), subnational intervention targeting can be refined to improve equity at the national level. For example, in units that could avert more than 10,000 combined DALYs under the counterfactual, most of the west sub-Saharan and DRC units would achieve this reduction by lowering malaria burden. Conversely, units in Ethiopia and northern Cameroon could experience dramatic declines in DALYs through reductions in DALYs from diarrhoea while north eastern Nigeria would benefit most from reductions in LRIs. Nigeria – the country with the highest combined burden on the continent and a population that includes 1/6 of all African children – represents a clear example of the impact heterogeneity can have. Of the 31.5 million (20.7–45.3) combined DALYs for Nigerian children in 2017, the elimination of spatial disparity in burden by bringing all units to at least the median rates for each disease would have averted 8.8 million (3.1–17.9; 28%) combined DALYs. Moreover, 308 (140–386) of the 775 units of Nigeria would have experienced a combined burden reduction of more than 10,000 DALYs. Had all units performed at the level of the best-performing unit in each year, in the west of Nigeria, the majority of the averted DALYs would have come from reductions in malaria (Fig. 3b ). In parts of the north-east, the reductions would be due to decreasing the high LRI burden while reductions would be due to decreasing the high malaria burden in parts of the northwest and central regions (Fig. 3b . ). Crucially, 4.5 million (1.7–8.5) combined DALYs would be averted in units where the reductions are needed across multiple causes (yellow and dark brown in Fig. 3b ), with 1.4 million (0.5–2.7) avertable combined DALYs occurring in units with almost identical relative levels of excess across all three causes (dark brown in Fig. 3b ). This counterfactual analysis makes clear that interventions that focused on bringing any single cause to its median rate across Nigeria would only address the burden for a subset of the population. Using Nigeria’s median performance as the baseline presents a more realistic view of what could be accomplished in a country based on prior experience; crucially, at least some of the wealthier, sub-optimally performing units stand to make improvements. Three of the most important causes of childhood disability and death in SSA (LRIs, diarrhoea, and malaria)—have substantial variation in the intensity of their combined burden as well as the relative composition of this burden. Our results demonstrate that within-country variation in combined burden manifests differently between countries with high simultaneous burden (as for CAR and Niger), while elsewhere the burden is more concentrated from a single cause (such as diarrhoea in Guinea-Bissau; 58% of combined burden). For many locations, particularly at subnational scales, the combined burden of death and disability from LRIs, diarrhoea, and malaria remains high, even as they reduced cause-specific burden. There has been substantial progress across SSA in reducing the disease burden from these causes since 2000 but these reductions have not been uniform. While some countries might benefit more than others from targeted interventions that focus on a single cause (such as malaria interventions in Burkina Faso or Sierra Leone), other countries are in need of general interventions across the entirety of the country (such as CAR). Alternately, some countries have a strong need for targeted interventions for one cause in one location, another cause in a second location, as well as general interventions in a third location (such as Nigeria). Understanding the combined burden in any given area can also be valuable in identifying the most effective interventions. For example, LRIs, the largest cause of under-5 burden in SSA among all causes, may be overlooked in these discussions because they are rarely the predominant cause of combined burden at a single location. Local decision-makers could also use these maps to assess whether strategies to deliver focused interventions, such as vaccines or mass drug administration, should be deployed differently in units where they would have the biggest impact (i.e., closing gaps in coverage or delivering the newly approved RTS,S malaria vaccine which is recommended only for high malaria burden regions [32] ). In 2017 alone, our findings show that more than 13 million (6.9–22.6) combined DALYs occurred in locations where the distribution of DALYs was divided similarly among the three causes. This represents a substantial burden to millions of children in SSA for whom integrated burden-reduction approaches will be required (Fig. 2b ). The examples we highlight of areas where decreases in burden over time have occurred for just one of these three dominant sources of death and disability for children under 5, can additionally provide motivation for treatment and prevention efforts that are at once more comprehensive in their scope and more precise in targeting specific locations of greatest need. Considering the overlapping risks related to childhood health (especially those related to LRIs, diarrhoea, and malaria), and the limited availability of resources to address such concerns, interventions that can decrease burden among multiple causes are ideal strategies, effective both in terms of burden reduction and cost [33] , [34] . Such interventions may span the range of maternal-child health including gender and education equity, maternal micro- and macronutrient fortification, promotion of exclusive breastfeeding, infant zinc and vitamin A supplementation, and complementary feeding programs [25] . Countries with exemplary reductions in under-5 mortality- including Ethiopia, Rwanda, and Senegal- introduced and empowered community or village health workers to connect children with healthcare and improve diagnosis and treatment of infectious diseases [35] . Detailed maps and estimates at subnational scales can show where disease burden is occurring with high precision. As we estimate more causes and risk factors of death and disability at the unit scale, the evidence-base for tailored integrated intervention packages that can reduce burden across multiple causes widens, increasing our capacity to target improvements in childhood health. Despite the advent of interventions that target U5M directly, such as the mass administration of azithromycin [36] , most intervention strategies are planned and delivered vertically. Here we show that as is true at the national level [26] , local variation in the major determinants of childhood disability and death will allow greater effectiveness in the geographical targeting of interventions, which can be further catalyzed by a universal platform for intervention delivery. A substantial focus of future research will be investigating how we can scale local analyses for a wider range of the principal determinants of U5M. First, more robust inferential methods must be created in order to identify the optimal interventions at local scales. Combining geo-referenced survey data and an inferential framework, while simultaneously modelling multiple causes in the same overarching scheme, will allow the description of the expected effect of different integrated intervention strategies from an assessment of the covariation of burden. From a methodological standpoint regarding the simultaneous modelling of multiple cases, care must be taken to balance model performance with inferentiality as many causes share the same underlying drivers. The ability to identify in detail the areas where prevention or intervention strategies have either been successful in reducing combined burden, or conversely reduced a cause-specific burden, can supply valuable case studies and suggest priorities for future interventions. Consistent with our counterfactual analysis, all regions with high burden would certainly benefit from universal improvements in health infrastructure, community case management, and in basic services like sanitation. Almost every country has the potential to improve their performance on at least one of these three diseases in at least some units, based on what has been achieved across all units already. In the absence of needed but costly and sweeping systematic changes in the health landscape across sub-Saharan Africa, the continued development of high-resolution maps of the distribution of disease burden across multiple causes of disease and disability can identify the areas where the greatest improvements in health can be achieved, with the fewest resources. In order to capitalise on these findings most effectively, local decision-makers could systematically analyse and apply this information in each unit across the African continent. We recognize that matching local policies and infrastructure to our findings would represent a substantial task, but we believe that this work can be used as a guide to focus discussions at the unit level as to which diseases are key to burden reduction. In the future, the availability of a comprehensive set of maps estimating mortality and DALYs for every major cause of under-5 mortality at the unit level, as well as additional efforts to co-map the most substantial contributors to the burden, have the potential to dramatically reduce the remaining preventable under-5 disease burden worldwide. Disability-adjusted life years (DALYs) The DALY [37] indicates health loss due to both nonfatal and fatal disease burden, calculated as the sum of years of life lost (YLLs) due to premature mortality and years lived with disability (YLDs). The YLL is based on remaining life expectancy when compared with a reference standard life table at age of death, and the YLD is calculated by multiplying the prevalence of a disease or injury and its main disabling outcomes by its weighted level of severity. As such, one DALY represents one year of healthy life lost. Note: when a location experiences a large amount of under-5 mortality, the average DALYs lost per year can exceed one even though every child who lives can only experience at most one DALY lost per year. Estimation of combined DALYs As discussed above, the individual cause-level spatio-temporally varying estimates of incidence, prevalence, and mortality for LRIs, diarrhoea, and malaria have been previously published [11] , [12] , [13] . Within each paper, the sources, model specifications and model validations are described in detail. Briefly, for malaria, data on incidence, prevalence, and mortality were combined through a number of modelling approaches to form internally consistent estimates. Chief amongst the modelling approaches was a Bayesian geostatistical technique that implemented an integrated nested Laplace approximation (INLA) model on the output of a stacked generalisation product using R-INLA v.20.01.29.9000 [38] , [39] . The INLA model accounted for spatial autocorrelation through the use of a Matérn covariance functional form and for temporal autocorrelation through the use of an autoregressive 1 (AR1) functional form. The INLA model allows both mean and uncertainty estimates to be created in terms of draws from a posterior distribution where individual draws represent a single possible spatiotemporal estimate. For both diarrhoea and LRIs, these estimates were based primarily on survey data assessing prevalence of the associated cause over the two weeks prior to the date of the survey. Again, both stacked generalisation and INLA were sequentially run to arrive at posterior estimates of spatiotemporal burden. For these two causes, a final step was conducted to align prevalence estimates with those of the Global Burden of Disease project [2] , [5] using logistic raking to ensure internally consistent estimates. The R project v.3.6.1 was used for all analyses. To create combined estimates of DALYs across the three causes, we first estimated YLLs from mortality and YLDs from incidence, both by draw in space-time. As the subnational estimates for each cause are designed to aggregate up to the country-level estimates (using population-weighted aggregation), and the YLLs and YLDs are constant multipliers of deaths and incidence, the mean value of the subnational YLLs and YLDs for each cause and country automatically agree with the corresponding mean country GBD estimate of the respective metric. We then estimated DALYs as above for each individual cause by posterior draw in space-time. As mentioned above, we assumed that the estimates for each cause are independent of one another, and as such to create draw-level estimates of the combined burden we added the draw-level estimates of each cause together. This created combined burden estimates in space and time with uncertainty. For aggregated estimates, we created population-weighted combined values again at the draw level. Population-based weights were derived from WorldPop estimates of under-5 population [40] . Maps were produced using ArcGIS Desktop 10.6. Calculation of annual rate of change (AROC) For each grid cell, we log-transformed the posterior mean prevalence estimates from each year from 2000 to 2017, \({{prev}}_{i,{yr}}^{l}\) , and determined the rate of change between each pair of adjacent years (beginning with yr=2001): 
    AROC_i, yr^l=prev_i, yr^l-prev_i, yr-1^l
 (1) Next, we took a weighted average AROC across the study period, placing more weight on more recent AROCs, and calculated grid-cell-level AROCs. Following Kinyoki et al. [41] , weight is defined as: 
    w_yr=(yr-2000)^γ/∑_2001^2017(yr-2000)^γ ,
 (2) in which different weights can be given to years across the study period by selecting the appropriate γ . For this analysis, we chose γ = 1 for a linear weighting scheme. We calculated grid-cell-level weighted-AROC as: 
    AROC_i=∑_2001^2017w_yrAROC_i, yr^l. (3) Finally, we calculated unit-level AROC values by taking population-weighted averages of all grid cells in a unit. Counterfactual analysis of averted DALYs We conducted a counterfactual analysis for each country independently. For each year, we identified the subnational unit with the lowest LRI burden, the unit with the lowest diarrhoea burden, and the unit with the lowest malaria burden. Our counterfactual scenario was based on setting every unit of that country at those minimum burden levels. As there are alternative counterfactuals that could be of interest (e.g., comparing each unit to the country average), we have provided the output as a table for others. Limitations Our work, as with any of this scope, comes with a number of limitations. First, we synthesised outputs of three independent modelling exercises into a single large analysis. Within each of those analyses there are limitations that translate to the overall work. In particular, the accuracy of any burden estimation is dependent on the quality and abundance of the data. Data coverage information in each of the three disease-specific models can be found in the supplementary material for each publication (page 26–54 [12] ; page 45–51 [11] ; page 37–42 [12] ) [11] , [12] , [13] . This analysis does not address any interactions between the pathogens that cause LRIs, diarrhoea, or malaria. Combining the limitations of data availability and potential overlap in cause-specific burden, we would expect the shared covariates used in the predictive statistical modelling to have similar direction of coefficients (for example, population density) leading to similar disease burden estimates in areas without data coverage. This analysis was intended to be a synthesis of each model, not a joint statistical analysis of each disease burden and so this type of correlation might be expected, especially given some regions within countries have more or fewer resources for public health efforts than others. Because we scaled the subnational disease burden estimates to the national level estimates from the Global Burden of Disease study, we expect there to be some countries with apparent higher or lower magnitude disease burden based on that scalar. Our counterfactual analysis was optimistic in the assumption that the best performing unit within a country is comparable to the rest of the units in the country. One reason for this optimistic approach was a desire to highlight that, for some locations, their substantial burden is actually average for their country. There are substantial differences between Figs. 3 in terms of observed burden and avertable burden under our counterfactual scenario and these differences specifically highlight the premise that some countries would benefit more from spatially-targeted interventions more than others. A deeper analysis that identifies more realistic strata of risk within a country based on similar disease ecology and then finds the best-performing unit within each strata as the baseline could create fairer comparisons and even more realistic counterfactual estimates. It is also important to note these causes also significantly contribute to DALYs in other age groups. There is a clear need for more detailed data on subnational variation of burden in older age groups as we do not expect the relative overlap of burdens in adults to perfectly match those of children. Reporting summary Further information on research design is available in the Nature Research Reporting Summary linked to this article.